Acidosis overrides oxygen deprivation to maintain mitochondrial function and cell survival Sustained cellular function and viability of high-energy demanding post-mitotic cells rely on the continuous supply of ATP. The utilization of mitochondrial oxidative phosphorylation for efficient ATP generation is a function of oxygen levels. As such, oxygen deprivation, in physiological or pathological settings, has profound effects on cell metabolism and survival. Here we show that mild extracellular acidosis, a physiological consequence of anaerobic metabolism, can reprogramme the mitochondrial metabolic pathway to preserve efficient ATP production regardless of oxygen levels. Acidosis initiates a rapid and reversible homeostatic programme that restructures mitochondria, by regulating mitochondrial dynamics and cristae architecture, to reconfigure mitochondrial efficiency, maintain mitochondrial function and cell survival. Preventing mitochondrial remodelling results in mitochondrial dysfunction, fragmentation and cell death. Our findings challenge the notion that oxygen availability is a key limiting factor in oxidative metabolism and brings forth the concept that mitochondrial morphology can dictate the bioenergetic status of post-mitotic cells. Long-term survival of post-mitotic cells, which have a limited regenerative capacity, is essential to ensure continued biological function of an organism. In recent years, it has become apparent that the decline of post-mitotic cells, during aging, neurodegenerative diseases and ischemic disorders, is generally associated with mitochondrial dysfunction [1] , [2] . Mitochondria are essential organelles for energy production, regulation of signalling cascades and cell death [3] . These organelles form a dynamic interconnecting network through continuous cycles of fission and fusion events [4] . The regulation of mitochondrial morphology is closely coupled to cell survival and metabolic adaptation during stress [5] , [6] , [7] . For example, aberrant mitochondrial fission has been observed in many disease and injury models and considered a key contributor to mitochondrial dysfunction and cell death [8] , [9] , [10] . In these settings, inhibition of mitochondrial fission or enhancing mitochondrial fusion restores cell viability [11] , [12] , [13] , [14] . These observations highlight the importance in the regulation of mitochondrial dynamics as a strategy to promote cellular survival. A common characteristic of high-energy-demanding post-mitotic cells, such as neurons, muscle and cardiomyocytes, is their dependence on a continuous supply of energy for sustained cellular function and viability. For this reason, contemporary eukaryotic cells are highly dependent on oxygen and functional mitochondria for the efficient generation of ATP through oxidative phosphorylation [15] , [16] . In this context, it can be appreciated how limitations in oxygen availability, or hypoxia, have profound physiological effects. Low oxygen levels cause major changes in mitochondrial structure and dynamics, ultimately leading to defective mitochondrial function, reduced ATP supply and activation of cell death pathways [17] , [18] , [19] . Importantly, a defective mitochondrial function induced by hypoxic stress is observed in diverse complex disorders such as type-2 diabetes mellitus, Alzheimer’s disease, cardiac and brain ischemia/reperfusion injury and tissue inflammation [17] . The fate of post-mitotic cells subjected to physiological or pathological settings of hypoxia is thus entirely reliant on their ability to respond and adapt to changing environments and stress conditions. Consequently, understanding oxygen sensing and response mechanisms in cells and tissues has been at the forefront of research for many years with the aim of exploiting adaptive strategies to promote cell survival. An essential and often neglected aspect of hypoxia is the accumulation of lactic acid as the end product of glycolysis. Excess H + ions resulting from an increased glycolytic rate are pumped outside the cell, inevitably causing acidification of the extracellular milieu. Physiological levels of acidosis in regions subjected to limited oxygen availability, such as the ischemic penumbra following a stroke, can range within the pH values of 6.0–6.5 depending on the severity of the insult [20] , [21] , [22] . A long-standing debate in biology is the effect of acidosis on cell survival. Although extracellular acidosis is historically viewed as a mere toxic byproduct of fermentation that is detrimental to cells, it is now clinically recognized as a protective agent when present at mild levels (pH 6.5 and above) [21] , [23] , [24] , [25] , [26] , [27] , [28] , [29] , [30] , [31] , [32] , [33] , [34] , [35] . In this regard, although several reports have clearly demonstrated the protective nature of mild acidosis, the underlying molecular mechanisms are still poorly understood. Furthermore, the role of mitochondria, being central to cell survival and death, has surprisingly never been addressed in this perspective. Here we show the unexpected observation that mild acidosis triggers massive morphological reorganization of mitochondria in post-mitotic cells, triggered by a dual programme that both activates fusion and cristae remodelling while inhibiting mitochondrial fragmentation. Activation of this reversible homeostatic programme reconfigures mitochondrial bioenergetics to allow for the persistence of efficient ATP production through oxidative phosphorylation despite oxygen limitations. Our work reveals a novel and physiological mechanism that can control the metabolic status of cells and protect mitochondrial-reliant post-mitotic cells following a hypoxic insult, by reprogramming mitochondrial morphology and functional efficiency. Acidosis triggers mitochondrial elongation during hypoxia As mitochondria are central in the cell death that is instigated during hypoxic stress, we investigated mitochondrial morphology in this setting. Cortical neurons were chosen for these experiments since they are a major population affected by hypoxic stress and thus represent a biologically relevant system for the study of adaptive mechanisms in post-mitotic cells. For our studies, we developed an in vitro model that mimics the physiological microenvironment found under hypoxic conditions, such as the penumbral region following an ischemic brain injury. This model recapitulates the low oxygen/glucose environment and takes into account that ischemic tissues or hypoxic cells normally acidify their extracellular milieu as a physiological consequence of anaerobic glycolysis. For this, a low glucose media was buffered in a manner to accommodate physiological acidification of the extracellular milieu when neurons are incubated at 1% O 2 (termed acidosis-permissive media (AP)). The control condition utilizes a low glucose media that maintains a stable neutral pH (pH 7.2) throughout experimentation (termed standard media (SD)). Mitochondria from cultured cortical neurons subjected to hypoxic conditions in a neutral pH environment had severely fragmented mitochondria as observed through immunofluorescence staining of the outer mitochondrial membrane protein Tom20 ( Fig. 1a and quantified in Fig. 1b ). Mitochondrial fragmentation was observed before signs of cell death or changes in neuronal morphology ( Supplementary Fig. 1 ). Unexpectedly, neurons subjected to hypoxia but allowed to undergo physiological extracellular acidification (measured pH post experiment was 6.5) exhibited massive mitochondrial elongation compared with control ( Fig. 1a and quantified in Fig. 1b ). Elongated mitochondria were observed in the cell body of cortical neurons and spanned along the axons ( Fig. 1c ). Mitochondrial elongation was also observed in cultured cerebellar granular neurons (CGNs; Fig. 1d,e ) and in vivo hippocampal slice preparations ( Fig. 1f,g ), as well as in differentiated C2C12 myotubes ( Supplementary Fig. 2 ), suggesting that this is a general phenomenon. Interestingly, acidosis-mediated mitochondrial elongation was not observed in proliferative cells, such as primary and transformed mouse embryonic fibroblast cells (MEF), C2C12 myoblasts, Cos7, HeLa and several cancer cell lines, including MCF-7, A549 and P19, suggesting that this response is unique to post-mitotic cells ( Supplementary Fig. 2 ). 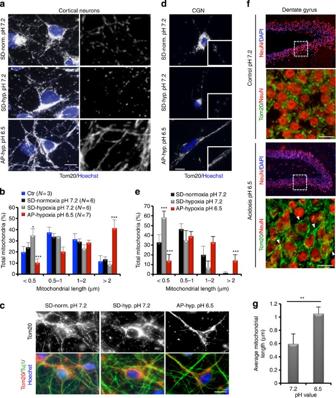Figure 1: Extracellular acidification restructures mitochondria in post-mitotic cells. (a) Representative confocal images of mitochondrial morphology in cultured cortical neurons following 18-h incubation at normoxic (Norm.) or hypoxic (Hyp.) conditions in SD or AP media. Mitochondria were visualized by Tom20 immunofluorescence. Panels on the right represent zoomed views of the mitochondria. (b) Mitochondrial length from (a) was quantified and binned into different length categories. Represented as mean and s.d. (nvalues indicated on graph). Ctr=control; represents neurons incubated in neurobasal media. (c) Representative images of mitochondrial morphology, revealed by Tom20 staining, in Tuj1+ cortical neurons at the indicated conditions. (dande) Mitochondrial morphology in cultured CGN after 18-h incubation at the indicated conditions. Insets in (d) are zoomed views of mitochondria. (e) Mean and s.d. (n=3) of mitochondrial length data in (d). (fandg) Mitochondrial morphology inex vivohippocampal slice preparations incubated in normoxia for 4 h at the indicated conditions. Neurons were immunostained with NeuN (neuronal-specific nuclear protein) and Tom20 (mitochondria). Panels showing Tom20/NeuN staining are zoomed views of the boxed area within the hippocampus. Arrowheads indicate elongated mitochondria. (g) Average mitochondrial length and s.d. were plotted for the indicated conditions. *P<0.05; **P<0.01; ***P<0.001 (Student’st-test). For all images scale=10 μm. Figure 1: Extracellular acidification restructures mitochondria in post-mitotic cells. ( a ) Representative confocal images of mitochondrial morphology in cultured cortical neurons following 18-h incubation at normoxic (Norm.) or hypoxic (Hyp.) conditions in SD or AP media. Mitochondria were visualized by Tom20 immunofluorescence. Panels on the right represent zoomed views of the mitochondria. ( b ) Mitochondrial length from ( a ) was quantified and binned into different length categories. Represented as mean and s.d. ( n values indicated on graph). Ctr=control; represents neurons incubated in neurobasal media. ( c ) Representative images of mitochondrial morphology, revealed by Tom20 staining, in Tuj1+ cortical neurons at the indicated conditions. ( d and e ) Mitochondrial morphology in cultured CGN after 18-h incubation at the indicated conditions. Insets in ( d ) are zoomed views of mitochondria. ( e ) Mean and s.d. ( n =3) of mitochondrial length data in ( d ). ( f and g ) Mitochondrial morphology in ex vivo hippocampal slice preparations incubated in normoxia for 4 h at the indicated conditions. Neurons were immunostained with NeuN (neuronal-specific nuclear protein) and Tom20 (mitochondria). Panels showing Tom20/NeuN staining are zoomed views of the boxed area within the hippocampus. Arrowheads indicate elongated mitochondria. ( g ) Average mitochondrial length and s.d. were plotted for the indicated conditions. * P <0.05; ** P <0.01; *** P <0.001 (Student’s t -test). For all images scale=10 μm. Full size image The acidosis-dependent alteration in mitochondrial morphology is pH-specific and elongation of mitochondria was only observed at a pH threshold value between 6.65 and 6.45 ( Fig. 2a,b and Supplementary Fig. 3 ), representing mildly acidic conditions as observed in physiological settings of hypoxic stress. In contrast, cells within a neutral (pH 7.2–6.8) or severely acidic (pH 6.0) extracellular environment during hypoxia exhibited significant mitochondrial fragmentation ( Fig. 2a,b and Supplementary Fig. 3 ). Acidosis-mediated mitochondrial elongation is a rapid process whereby the onset of elongation occurred at about 3-h post-treatment ( Fig. 2c,d and Supplementary Fig. 4 ). This opposed the hypoxia-mediated mitochondrial fragmentation that occurs in neutral conditions beginning 3 h following treatment ( Fig. 2c and Supplementary Fig. 4 ). In addition, although acidosis generally occurs as a consequence of increased glycolysis during limited oxygen availability, its effect on mitochondrial morphology was in fact independent of oxygen. Incubation of cortical neurons in media set to pH 6.5 in the presence of oxygen (normoxia) resulted in a significant increase in mitochondrial length compared with control ( Fig. 2e ). To further confirm the direct affect of acidosis on mitochondrial length, the contribution of low glucose levels in the experimental paradigm, which represents a more physiologically relevant setting, was assessed. The effect of acidosis on mitochondrial length was not a consequence of decreased glucose availability since mitochondrial elongation persisted in the presence of high glucose levels ( Fig. 2f and Supplementary Fig. 5 ). Thus, mitochondrial elongation in these settings is directly mediated by acidosis and is not a consequence of an induced starvation response. This is supported by the observation that the limited glucose availability in these experiments was not sufficient to activate autophagy ( Supplementary Fig. 6 ) such as that observed during complete glucose starvation, where there is a marked increase in LC3II, degradation of p62 and loss of outer membrane Tom20 due to mitophagy ( Supplementary Fig. 6 ). These results demonstrate that acidosis alone is sufficient to promote mitochondrial elongation. Acidosis-driven elongation is also a reversible process. Mitochondria remain elongated regardless of oxygen levels, confirming that this process is oxygen-independent ( Fig. 2g,h and Supplementary Fig. 7 ). However, mitochondria revert back to a fragmented phenotype following neutralization of the extracellular pH both under hypoxic or reoxygenation conditions ( Fig. 2g,h and Supplementary Fig. 7 ). In fact, the level of fragmentation following reoxygenation in a neutral context was very rapid (within 30 min) and was quite severe ( Fig. 2h and Supplementary Fig. 7 ). In order to gain insight as to how extracellular acidosis can relay an intracellular signal to modify mitochondrial morphology, pH changes within the intracellular environment were examined. Analysis of intracellular pH changes using the ratiometric fluorescent indicator BCECF-AM ( Supplementary Fig. 8a ) showed that a decrease in extracellular pH as used in our studies (pH 6.5) was sufficient to cause a reduction in intracellular pH ( Supplementary Fig. 8b ) and is consistent with previous reports showing that intracellular pH can be modified by the extracellular milieu [36] , [37] . Furthermore, neutralization of the intracellular pH using the Na+/H+ exchanger Monensin ( Supplementary Fig. 8c ) rapidly reverses the mitochondrial elongation phenotype that was instigated by extracellular acidosis ( Fig. 2i and Supplementary Fig. 8d,e ). Together, these results demonstrate a pH-dependent regulation of mitochondrial morphology that is oxygen- and glucose-independent and is reversible. 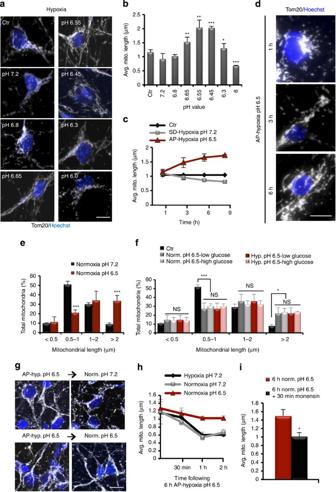Figure 2: Acidosis-mediated mitochondrial elongation is pH-specific, rapid, reversible and O2- and glucose-independent. (a) Representative confocal images of mitochondrial morphology in cultured cortical neurons following incubation at fixed pH values in hypoxia. Ctr=control; represents neurons incubated in neurobasal media. (b) Average mitochondrial length and s.d. (n=3) were plotted for the indicated pH values. (c) Average mitochondrial length and s.d. (n=3) over time at indicated conditions. (d) Immunofluorescence of Tom20 (mitochondria) showing the change in mitochondrial length in cortical neurons by physiological acidosis at the indicated times. (e) Mean and s.d. (n=3) of mitochondrial length distribution during normoxic conditions at indicated pH values for 6 h. (f) Mean and s.d. (n=3) of mitochondrial length distribution during normoxic or hypoxic conditions in the presence of low (5.5 mM) or high (25 mM) glucose levels for 6 h. (gandh) Analysis of mitochondrial morphology after 6-h incubation in AP-Hypoxia pH 6.5 and following reoxygenation at the indicated pH values. (h) Graph of the change in average mitochondrial length (s.d.,n=3) at the indicated conditions following a 6-h incubation in AP-Hypoxia pH 6.5. (i) Average mitochondrial length and s.d. (n=3) were plotted for the indicated conditions. ns=not significant, *P<0.05; **P<0.01; ***P<0.001 (Student’st-test). For all images scale=10 μm. Figure 2: Acidosis-mediated mitochondrial elongation is pH-specific, rapid, reversible and O 2 - and glucose-independent. ( a ) Representative confocal images of mitochondrial morphology in cultured cortical neurons following incubation at fixed pH values in hypoxia. Ctr=control; represents neurons incubated in neurobasal media. ( b ) Average mitochondrial length and s.d. ( n =3) were plotted for the indicated pH values. ( c ) Average mitochondrial length and s.d. ( n =3) over time at indicated conditions. ( d ) Immunofluorescence of Tom20 (mitochondria) showing the change in mitochondrial length in cortical neurons by physiological acidosis at the indicated times. ( e ) Mean and s.d. ( n =3) of mitochondrial length distribution during normoxic conditions at indicated pH values for 6 h. ( f ) Mean and s.d. ( n =3) of mitochondrial length distribution during normoxic or hypoxic conditions in the presence of low (5.5 mM) or high (25 mM) glucose levels for 6 h. ( g and h ) Analysis of mitochondrial morphology after 6-h incubation in AP-Hypoxia pH 6.5 and following reoxygenation at the indicated pH values. ( h ) Graph of the change in average mitochondrial length (s.d., n =3) at the indicated conditions following a 6-h incubation in AP-Hypoxia pH 6.5. ( i ) Average mitochondrial length and s.d. ( n =3) were plotted for the indicated conditions. ns=not significant, * P <0.05; ** P <0.01; *** P <0.001 (Student’s t -test). For all images scale=10 μm. Full size image Acidosis inhibits DRP1-mediated mitochondrial fission Mitochondrial fragmentation is a prominent phenotype during hypoxic stress conditions as observed here ( Figs 1a,b and 2c ) and in previous studies [19] , [38] , [39] . However, physiological acidification appears to prevent hypoxia-induced mitochondrial fragmentation. An essential component of the mitochondrial fission machinery, the dynamin protein DRP1, is a cytosolic factor that is recruited to mitochondria upon activation [40] . As expected, localization analysis of endogenous DRP1 showed a pronounced increase in mitochondrial-specific DRP1 foci during hypoxia-neutral conditions that correlate with the observed increase in fragmentation ( Fig. 3a,b ). Interestingly, a decrease in the number of DRP1 foci per unit length of mitochondria was observed during acidosis ( Fig. 3a,b ). A decline in mitochondrial DRP1 during acidosis was not due to changes in total cellular protein expression of DRP1 ( Fig. 3c ) but was reminiscent of the decreased number of mitochondrial DRP1 foci observed in the presence of the selective inhibitor of DRP1-mediated mitochondrial fission, Mdivi-1(ref. 41 ; Fig. 3d ). Analysis of DRP1 protein interactions revealed that in cultured cortical neurons DRP1 associates with Fis1 but not Mff, two previously identified DRP1-binding proteins ( Supplementary Fig. 9a ) [42] . Furthermore, immunoprecipitation of endogenous DRP1 at the onset of mitochondrial elongation by acidosis revealed a decreased level of interaction between DRP1 and Fis1, a mitochondrial DRP1-binding protein important for DRP1 recruitment and fission [42] , [43] . The decrease in DRP1–Fis1 interaction was similar to what is observed following treatment with forskolin, an inhibitor of fission through its activation of PKA-mediated phosphorylation and inhibition of DRP1 recruitment to mitochondria ( Fig. 3e and Supplementary Fig. 9b,d ). These data suggest that acidosis inhibits DRP1-mediated fission during hypoxia. Although PKA-dependent phosphorylation at Ser637 represents a major regulatory sight for DRP1 activation [44] , we did not observe a change in the phosphorylation status of DRP1 at Ser637. Moreover, inhibition of the PKA pathway did not affect acidosis-mediated mitochondrial elongation nor did activation of this pathway affects mitochondrial morphology during hypoxia ( Supplementary Fig. 9b,d ). Furthermore, the phosphorylation status of DRP1 at Ser616, a common target of DRP1 regulation during oxidative stress [45] , was not altered at the time point where mitochondrial elongation is observed ( Supplementary Fig. 9c ). Thus, mild acidosis prevents mitochondrial fragmentation under hypoxic conditions through the PKA and CDK1/PKCδ-independent regulation of DRP1 activation and recruitment to mitochondria. 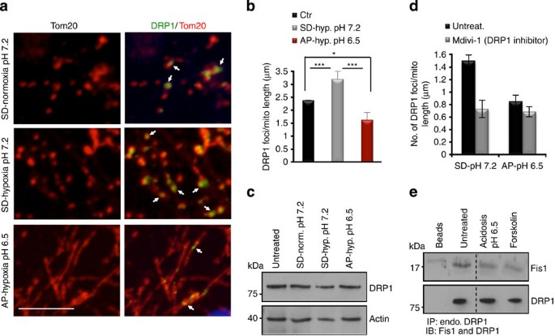Figure 3: Mild acidosis inhibits DRP1-mediated mitochondrial fission. (a) Colocalization of DRP1 foci at mitochondria by immunofluorescence of DRP1 and Tom20 in cortical neurons using confocal imaging. Arrows show DRP1 foci localized at mitochondria. Scale=5 μm. (b) Quantification of the number of DRP1 foci colocalized to mitochondria and represented as mean and s.d. (n=3). (c) Western blot of the indicated proteins from whole cell lysates of cultured cortical neurons following 6-h incubation at the indicated conditions. (d) Quantification of the number of DRP1 foci colocalized to mitochondria following 6-h hypoxic incubation in SD or AP media in the presence or absence of the fission inhibitor Mdivi-1. (e) Western blot of indicated proteins following incubation for 3 h at the indicated conditions and immunoprecipitation of endogenous (endo.) DRP1 using anti-DRP1 antibody. Figure 3: Mild acidosis inhibits DRP1-mediated mitochondrial fission. ( a ) Colocalization of DRP1 foci at mitochondria by immunofluorescence of DRP1 and Tom20 in cortical neurons using confocal imaging. Arrows show DRP1 foci localized at mitochondria. Scale=5 μm. ( b ) Quantification of the number of DRP1 foci colocalized to mitochondria and represented as mean and s.d. ( n =3). ( c ) Western blot of the indicated proteins from whole cell lysates of cultured cortical neurons following 6-h incubation at the indicated conditions. ( d ) Quantification of the number of DRP1 foci colocalized to mitochondria following 6-h hypoxic incubation in SD or AP media in the presence or absence of the fission inhibitor Mdivi-1. ( e ) Western blot of indicated proteins following incubation for 3 h at the indicated conditions and immunoprecipitation of endogenous (endo.) DRP1 using anti-DRP1 antibody. Full size image Mitochondrial fusion by acidosis depends on the SIMH pathway The degree and rate of elongation observed during acidosis suggested the possibility of a pH-dependent enhancement in mitochondrial fusion activity, in addition to suppression of the fission pathway. This was tested in live neurons, infected with a mitochondrial matrix targeted photo-activatable green-fluorescent protein (GFP) lentivirus (PA-Oct-GFP), following 3 h of incubation at pH 7.2 or 6.5 under normoxic conditions, representing the onset of elongation in the absence of hypoxia-induced fission. The rate of dilution and spread of the photo-converted GFP molecules are used as a measure of fusion activity. Time-lapse imaging of the activated mitochondrial GFP signal demonstrated an increase in mitochondrial fusion in neurons subjected to mild acidosis ( Fig. 4a,b and Supplementary Fig. 10 ). Examination of mitochondrial mass further confirmed that mitochondrial elongation during acidosis is a result of enhanced fusion activity rather than increased mitochondrial biogenesis since the levels of resident mitochondrial proteins HSP70 and VDAC were unchanged ( Fig. 4c ). Mitochondrial elongation during acidosis does not appear to be activated through increased expression levels of core fusion proteins OPA1 and MFN1/2 (refs 46 , 47 , 48 ; Fig. 4d ). Moreover, addition of the protein synthesis inhibitor cycloheximide did not prevent acidosis-mediated mitochondrial elongation or significantly alter mitochondrial length during control conditions, suggesting that acidosis may regulate mitochondrial dynamics at the post-translational level ( Supplementary Fig. 11 ). To further decipher the molecular mechanism enabling enhanced fusion activity, we examined the possibility that acidosis activates the stress-induced mitochondrial hyperfusion (SIMH) pathway [7] . We found that removal of the key molecular components of the mitochondrial fusion machinery and the SIMH pathway, OPA1, MFN1 and SLP2, rendered neurons unresponsive to acidosis-induced mitochondrial elongation in normoxia ( Fig. 4e,f ). Together, these data demonstrate that mild acidosis enhances mitochondrial fusion, requires an intact fusion machinery and suggests a specific role for the SIMH pathway in the hyperfusion observed by mild acidosis during hypoxic stress. 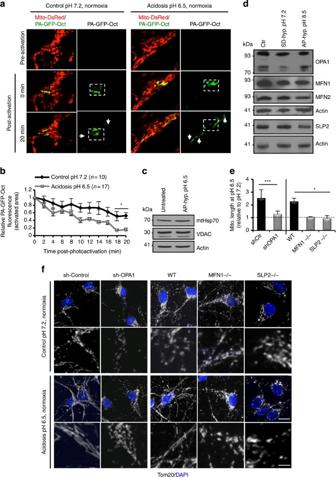Figure 4: Mild acidosis regulates mitochondrial dynamics. (a) Representative images of mitochondrial fusion over time (indicated in minutes) following activation of exogenously expressed PA-GFP-Oct. Boxes indicate photo-activated regions and arrows indicate spread of the GFP signal within mitochondria (revealed by exogenous expression of Mito-DsRed). (b) Quantification of mitochondrial fusion in cortical neurons as a loss of GFP fluorescence in the activated region. Data represent the mean and s.d. ofn=10 (control) andn=17 (experimental) from three independent experiments. (candd) Western blot of the indicated proteins from whole-cell lysates of cortical neurons incubated for 6 h at the indicated conditions. Asterisk indicates s-OPA1. (e) Mean and s.d. (n=3) of mitochondrial length during acidosis, of the indicated genotypes, relative to control conditions. (f) Representative images of mitochondrial morphology from cortical neurons of the indicated genotypes following 6-h incubation in MES-buffered media at the indicated conditions. Bottom panel of each condition is a zoom view of mitochondria. Scale=10 μm. *P<0.05; ***P<0.001 (Student’st-test). Figure 4: Mild acidosis regulates mitochondrial dynamics. ( a ) Representative images of mitochondrial fusion over time (indicated in minutes) following activation of exogenously expressed PA-GFP-Oct. Boxes indicate photo-activated regions and arrows indicate spread of the GFP signal within mitochondria (revealed by exogenous expression of Mito-DsRed). ( b ) Quantification of mitochondrial fusion in cortical neurons as a loss of GFP fluorescence in the activated region. Data represent the mean and s.d. of n =10 (control) and n =17 (experimental) from three independent experiments. ( c and d ) Western blot of the indicated proteins from whole-cell lysates of cortical neurons incubated for 6 h at the indicated conditions. Asterisk indicates s-OPA1. ( e ) Mean and s.d. ( n =3) of mitochondrial length during acidosis, of the indicated genotypes, relative to control conditions. ( f ) Representative images of mitochondrial morphology from cortical neurons of the indicated genotypes following 6-h incubation in MES-buffered media at the indicated conditions. Bottom panel of each condition is a zoom view of mitochondria. Scale=10 μm. * P <0.05; *** P <0.001 (Student’s t -test). Full size image Acidosis regulates cristae remodelling during stress The internal structures of mitochondria, the cristae, are also dynamic and can undergo OPA1-dependent remodelling during stress conditions [49] , [50] . OPA1 oligomeric complexes, consisting of both membrane-bound long (l-OPA1) and soluble short forms (s-OPA1) of OPA1 in the intermembrane space, have been associated with inner membrane morphology, tightness of the cristae junctions, as well as sequestration of Cytochrome c (Cyt C ) within the cristae [46] , [49] , [51] , [52] . We found that the relative amount of s-OPA1 was altered following 6 h of hypoxic treatment ( Fig. 4d ) and OPA1-specific oligomeric complexes were disrupted as early as 1 h after treatment ( Fig. 5a and Supplementary Fig. 12 ). However, a mild decrease in the extracellular pH during hypoxia rescued both the levels of s-OPA1 and OPA1 oligomeric complexes ( Figs 4d and 5a ). Acidosis also increased OPA1 oligomeric complexes under normoxic conditions ( Fig. 5b ). This suggested that acidosis not only changes mitochondrial length but it may also alter cristae morphology. Examination of mitochondrial ultrastructure using transmission electron microscopy (TEM) revealed that mitochondrial ultrastructure, which is severely disrupted during hypoxia, was preserved by acidosis ( Fig. 5c–e ). During hypoxia-neutral conditions, where aberrant mitochondrial fragmentation is observed, there is a severe disruption of mitochondrial ultrastructure leading to a significant increase in cristae diameter as well as a reduction in cristae number ( Fig. 5c–e ). More importantly, a mild decrease in the pH during hypoxia not only rescued this defect but also resulted in a significant tightness of the cristae diameter and increased cristae number, relative to control ( Fig. 5c–e ). These data suggest a role for acidosis in cristae maintenance and remodelling. This was further confirmed through an indirect examination of cristae remodelling by measuring the degree of Cyt C release following an apoptotic stimulus, which can provide information related to the tightness of the cristae junctions [49] , [53] . Treatment of neurons with Camptothecin (CPT), a DNA-damaging agent that triggers the apoptotic cell death pathway, revealed that mitochondrial restructuring by acidosis renders cells resistant to Cyt C release ( Fig. 5f,g ), in the presence of apoptosis signalling as indicated by BAX activation ( Supplementary Fig. 13 ). Together, these data demonstrate that mild acidosis modulates mitochondrial dynamics as well as cristae architecture. Furthermore, these data suggest that acidosis prevents the intramitochondrial remodelling, as a result of OPA1 oligomer destabilization, that is associated with mitochondrial fragmentation and cell death signalling. 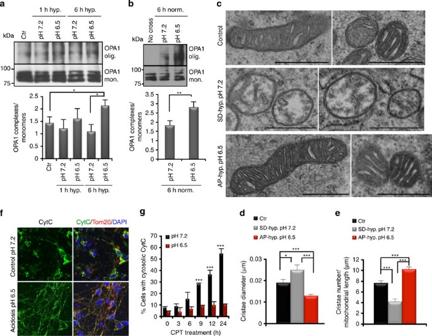Figure 5: Mild acidosis regulates cristae architecture. (a,b) Western blot of OPA1 oligomers and monomers from lysates of BMH crosslinking in live cortical neurons at the indicated conditions. OPA1 western blot has been spliced to better clarify where monomeric and oligomerized Opa1 appear. Graphs represent the mean and s.d. (n=3) quantification of OPA1 oligomer:monomer ratio. (c–e) Representative EM images of mitochondrial ultrastructure following 6-h incubation at the indicated conditions. Scale=500 nm. Graphs in (d,e) represent mean and s.e.m (n=10) for quantification of cristae diameter and cristae number. Ctr=control represents neurons incubated in neurobasal media. (f,g) Representative images and quantification (mean and s.d.,n=4) of CytC localization following CPT treatment in MES-buffered media at pH 7.2 or 6.5 in normoxia. *P<0.05; **P<0.01; ***P<0.001 (Student’st-test). Figure 5: Mild acidosis regulates cristae architecture. ( a , b ) Western blot of OPA1 oligomers and monomers from lysates of BMH crosslinking in live cortical neurons at the indicated conditions. OPA1 western blot has been spliced to better clarify where monomeric and oligomerized Opa1 appear. Graphs represent the mean and s.d. ( n =3) quantification of OPA1 oligomer:monomer ratio. ( c – e ) Representative EM images of mitochondrial ultrastructure following 6-h incubation at the indicated conditions. Scale=500 nm. Graphs in ( d , e ) represent mean and s.e.m ( n =10) for quantification of cristae diameter and cristae number. Ctr=control represents neurons incubated in neurobasal media. ( f , g ) Representative images and quantification (mean and s.d., n =4) of CytC localization following CPT treatment in MES-buffered media at pH 7.2 or 6.5 in normoxia. * P <0.05; ** P <0.01; *** P <0.001 (Student’s t -test). Full size image Mitochondrial restructuring protects cells in hypoxia Several studies have demonstrated the protective effect of mild acidosis during ischemic conditions. Importantly, this observation was recapitulated in our model of ischemia. A significant increase in cell death is observed in hypoxia under neutral conditions; however, a physiological decrease in the extracellular pH (pH 6.5) protects neurons from death ( Fig. 6a ). Interestingly, acidosis rendered neurons resistant to other damaging agents such as CPT ( Fig. 6b ), suggesting that cells subjected to mild changes in extracellular pH can sustain survival under different modes of stress. The observation that mild acidosis in our system also promotes mitochondrial remodelling suggests that this may be the underlying mechanism of cellular protection previously observed at similar pH levels. To confirm this hypothesis, we tested neuronal survival during hypoxia–acidosis where we prevented the impact of acidosis on mitochondrial dynamics. The protective effect of acidosis was reversed in the absence of the essential fusion machinery. Acute RNA interference-mediated loss of OPA1 expression or genetic ablation of MFN1 prevented acidosis-mediated mitochondrial elongation ( Fig. 4e,f ) and was sufficient to increase cell death during hypoxia even in the presence of acidosis ( Fig. 6c,d ). Moreover, overexpression of the mitochondrial fission protein DRP1, in wild-type neurons, resulted in a significant increase in cell death during hypoxia–acidosis ( Fig. 6e ). These data demonstrate that the restructuring of mitochondria during stress is a major player in the protective effect of mild acidosis. 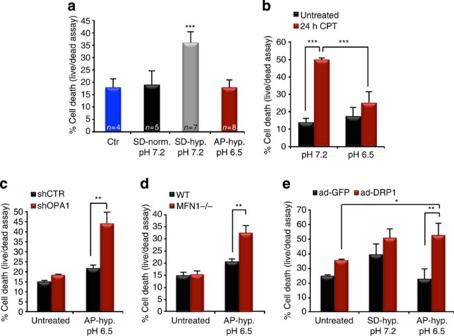Figure 6: Acidosis-mediated mitochondrial remodelling protects neurons from cell death during hypoxic stress. (a) Quantification of cell death of cortical neurons as mean and s.d. (nvalues indicate independent experiments) following 30-h incubation in SD or AP media at the indicated conditions. (b) Mean and s.d. (n=3) of neuronal cell death analysis following 24-h treatment with CPT in MES-buffered media at pH 7.2 or 6.5 in normoxia. (c) Quantification of cell death in neurons infected with lentivirus encoding a scrambled (shCTR) or OPA1-specific (shOPA1) shRNA following 30 h in SD or AP media at the indicated conditions (mean and s.d.,n=3). (d) Mean and s.d. (n=4) of cell death quantification in WT (wild-type) or MFN1-deficient (MFN1−/−) cortical neurons following 30-h incubation in SD or AP media at the indicated conditions. (e) Quantification of cell death in neurons infected with adenovirus-encoding GFP or DRP1-YFP following 30-h incubation in SD or AP media at the indicated conditions (mean and s.d.,n=3). *P<0.05; **P<0.01; ***P<0.001 (Student’st-test). Figure 6: Acidosis-mediated mitochondrial remodelling protects neurons from cell death during hypoxic stress. ( a ) Quantification of cell death of cortical neurons as mean and s.d. ( n values indicate independent experiments) following 30-h incubation in SD or AP media at the indicated conditions. ( b ) Mean and s.d. ( n =3) of neuronal cell death analysis following 24-h treatment with CPT in MES-buffered media at pH 7.2 or 6.5 in normoxia. ( c ) Quantification of cell death in neurons infected with lentivirus encoding a scrambled (shCTR) or OPA1-specific (shOPA1) shRNA following 30 h in SD or AP media at the indicated conditions (mean and s.d., n =3). ( d ) Mean and s.d. ( n =4) of cell death quantification in WT (wild-type) or MFN1-deficient (MFN1−/−) cortical neurons following 30-h incubation in SD or AP media at the indicated conditions. ( e ) Quantification of cell death in neurons infected with adenovirus-encoding GFP or DRP1-YFP following 30-h incubation in SD or AP media at the indicated conditions (mean and s.d., n =3). * P <0.05; ** P <0.01; *** P <0.001 (Student’s t -test). Full size image Reprogrammed mitochondria maintain ATP production in hypoxia A prominent response to cellular hypoxic stress is mitochondrial fragmentation, and loss of mitochondrial membrane potential and dysfunction [17] , [19] . Since acidosis prevents hypoxia-induced mitochondrial fragmentation and cell death, we wanted to investigate the status of mitochondrial integrity and function. We found that mild acidosis maintains mitochondrial membrane potential during hypoxia ( Fig. 7a , and Supplementary Fig. 14 ). Maintenance of mitochondrial membrane potential requires a protonmotive force that is generated by the electron transport chain through respiration or, in pathological situations, by ATP hydrolysis via the F 1 F 0 -ATPase (ATP synthase). A highly polarized membrane potential suggests that either mitochondrial respiratory function was preserved by mild acidosis or that the membrane potential was maintained by the reversal of the ATP synthase, which would result in ATP consumption. Interestingly, total ATP levels were sustained for an extended period in hypoxia if cells underwent physiological acidification ( Fig. 7b ), suggesting that ATP hydrolysis by the ATP synthase was not a central contributing factor in maintaining membrane potential. 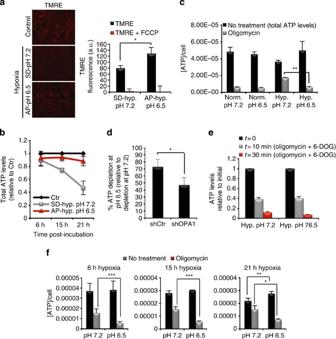Figure 7: Acidosis maintains mitochondrial function during hypoxic stress. (a) TMRE staining and quantification of fluorescence intensity following 18-h incubation in SD or AP media in hypoxia. Mean and s.d. (n=3 from three independent experiments). The uncoupler FCCP, which dissipates the membrane potential, is used to show specificity of the measured TMRE fluorescence. (b) Total ATP levels relative to normoxic control (in black). Mean and s.d. (n=5). (c) Total ATP concentration per cell at steady state (black) and after 1-h oligomycin treatment (grey) following 6 h of treatment at the indicated conditions. Mean and s.d. (n=3 replicates from six independent experiments). (d) Quantification of the amount of ATP depletion following 1-h oligomycin treatment in cortical neurons infected with lentivirus encoding a scrambled control (shCtr) or OPA1-specific shRNA (shOPA1). Mean and s.d. (n=3 replicates from three independent experiments). (e) ATP levels per cell relative to initial values (black) following oligomycin and 6-DOG treatment. Mean and s.d. (n=3 replicates from three independent experiments). (f) Total ATP levels per cell at steady state (black) and after 1-h oligomycin treatment (grey). Graphs represent mean and s.d. ofn=3 replicates from six independent experiments. *P<0.05; **P<0.01; ***P<0.001 (Student’st-test). Figure 7: Acidosis maintains mitochondrial function during hypoxic stress. ( a ) TMRE staining and quantification of fluorescence intensity following 18-h incubation in SD or AP media in hypoxia. Mean and s.d. ( n =3 from three independent experiments). The uncoupler FCCP, which dissipates the membrane potential, is used to show specificity of the measured TMRE fluorescence. ( b ) Total ATP levels relative to normoxic control (in black). Mean and s.d. ( n =5). ( c ) Total ATP concentration per cell at steady state (black) and after 1-h oligomycin treatment (grey) following 6 h of treatment at the indicated conditions. Mean and s.d. ( n =3 replicates from six independent experiments). ( d ) Quantification of the amount of ATP depletion following 1-h oligomycin treatment in cortical neurons infected with lentivirus encoding a scrambled control (shCtr) or OPA1-specific shRNA (shOPA1). Mean and s.d. ( n =3 replicates from three independent experiments). ( e ) ATP levels per cell relative to initial values (black) following oligomycin and 6-DOG treatment. Mean and s.d. ( n =3 replicates from three independent experiments). ( f ) Total ATP levels per cell at steady state (black) and after 1-h oligomycin treatment (grey). Graphs represent mean and s.d. of n =3 replicates from six independent experiments. * P <0.05; ** P <0.01; *** P <0.001 (Student’s t -test). Full size image It is well established that mitochondrial function and the generation of ATP through oxidative phosphorylation (OXPHOS) is impaired during hypoxic conditions, causing cells to shift to anaerobic glycolysis [54] . Although this shift in metabolism is important for cell survival during acute hypoxic stress, glycolysis represents a much less efficient mode of ATP production, and over the long run it is reasonable to conceive how this can pose an energy deficit in high-energy-demanding cells such as neurons. The remodelling of mitochondria, as well as maintained membrane potential and ATP levels by acidosis, led us to postulate that acidosis may also preserve mitochondrial function during hypoxic conditions. Intriguingly, we found that addition of oligomycin, an ATP synthase inhibitor that blocks mitochondrial ATP production, resulted in a significant depletion, of ~90%, in total ATP levels during hypoxia–acidosis conditions, to the same extent as that observed during normoxia (at pH 7.2 and 6.5; Fig. 7c ). This is in contrast to what is observed under hypoxia-neutral conditions whereby oligomycin treatment following short-term hypoxia (6 h) results in only about 50% decrease in ATP levels, suggesting the use of a non-mitochondrial ATP production pathway (that is, glycolysis). Preventing mitochondrial fusion and disrupting cristae structure during acidosis, through acute loss of OPA1 expression, resulted in decreased oligomycin-sensitive ATP depletion at pH 6.5 ( Fig. 7d ). The increased level of ATP depletion in wild-type neurons, observed in the presence of oligomycin during acidosis, was not due to an elevation in ATP utilization since arrest of both ATP production pathways using 6-deoxyglucose (6-DOG; glycolysis inhibitor) and oligomycin showed a similar rate of ATP consumption over time during hypoxia at pH 7.2 and 6.5 ( Fig. 7e ). Given that an increase in consumption cannot account for the significant depletion of ATP in the presence of oligomycin, this suggests that cells in acidosis rely less on the glycolytic ATP generation pathway and supports the idea that acidosis preserves mitochondrial function and sustains OXPHOS during hypoxia. This observation was quite surprising considering that oxygen availability is historically viewed as a limiting factor for mitochondrial ATP generation through mitochondrial respiration. More importantly, a pH-dependent shift in the bioenergetic status of neurons was observed over time, whereby cells in hypoxia at pH 7.2 relied increasingly on oligomycin-insensitive ATP production (that is, glycolysis) while neurons allowed to undergo physiological acidification relied on mitochondrial-dependent ATP production ( Fig. 7f ). Thus, acidosis sustains efficient mitochondrial ATP production during prolonged hypoxia ( Fig. 7f ). An alteration in the metabolic profile of cells in hypoxia–acidosis implies an adaptation of the electron transport chain (ETC) components to maximize mitochondrial efficiency during limited oxygen availability. Several studies have reported the adverse effect of hypoxia on the expression and activity of ETC complexes as well as supercomplex disassembly [55] , [56] . Expression analysis of subunits encompassing the ETC complexes during acute hypoxia revealed maintained expression of Complex I subunit NDUFA9 as well as ATP synthase subunit ATP5a by mild acidosis ( Supplementary Fig. 15 ). Blue native PAGE (BN-PAGE) analysis of the respiratory chain complexes showed a destabilization of the monomeric ATP synthase multiprotein complex during hypoxia, which is rescued by acidosis ( Fig. 8a,b ). Only a minor proportion of the ATP synthase is present in its dimeric form in neurons used during our experiments ( Fig. 8c and Supplementary Fig. 16 ). Nonetheless, longer exposure of BN-PAGE from whole cells or BN-PAGE performed on isolated mitochondria revealed a higher molecular weight band corresponding to dimeric forms of the ATP synthase predominantly in hypoxia–acidosis conditions ( Fig. 8c,d and Supplementary Fig. 16 ), indicating a distinct rise in the stability of the enzyme superassembly. The individual multiprotein complexes of the ETC can further associate into supercomplexes, known as respirasomes [57] , [58] . It has been proposed that supercomplex assembly could stabilize the single complexes, enhance the electron flow between complexes and limit generation of oxygen radicals [59] , [60] , [61] , [62] , [63] . In addition, a distinct role for cristae shape has been recently shown to affect supercomplex assembly and respiratory efficiency [64] . Examination of higher order respiratory complex assembly by BN-PAGE showed a distinct reorganization of Complex I-containing supercomplexes by acidosis regardless of oxygen levels ( Fig. 8e ), resulting in loss of monomeric complex I and enhanced supercomplex assembly (complex I supercomplex:monomer ratio; Fig. 8h ), as well as an increase in the relative levels ( Fig. 8f ). Detailed analysis of the respiratory supercomplexes showed maintained assembly of Complexes 1, III and IV into supercomplexes in the presence of acidosis during hypoxic conditions ( Fig. 8g,h ). We hypothesized that the acidosis-mediated changes to the OXPHOS complexes would be accompanied by an enhancement in the respiratory capacity of mitochondria. To test this hypothesis, the bioenergetic profile of mitochondria was assessed in intact neurons exposed to normoxic conditions at pH 7.2 and 6.5. First, basal cellular and mitochondrial oxygen consumption rate (OCR) was similar in both conditions ( Fig. 8i,j ). Next, the mitochondrial respiration capacity was determined using the uncoupler FCCP, which stimulates maximal mitochondrial respiration by dissipating the mitochondrial membrane potential. We found that acidosis significantly enhances the ability of mitochondria to increase their maximal respiratory capacity ( Fig. 8i,j ). In addition, analysis of mitochondrial reserve capacity, which signifies the ability of mitochondria to further engage in the production of ATP through OXPHOS, revealed a significant increase at pH 6.5 ( Fig. 8i,j ). These data coupled with data obtained from ATP studies provide evidence that acidosis maintains mitochondrial function during hypoxic stress. This is achieved through an adaptive reprogramming of mitochondrial respiratory efficiency that occurs as a result of changes in the mitochondrial ultrastructure and cristae shape, respiratory supercomplex assembly and maintenance of monomeric ATP synthase. 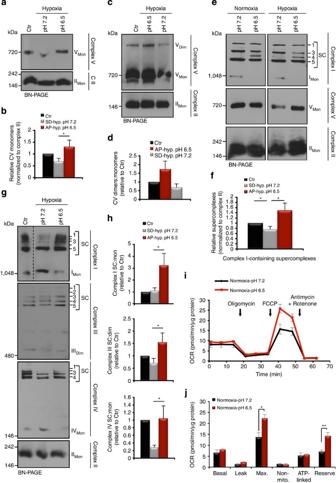Figure 8: Acidosis instigates an adaptive reprogramming of mitochondrial respiratory efficiency. (a–d) Representative BN-PAGE of Complex V (ATP synthase) (a) monomers (whole cells) and (c) dimers (isolated mitochondria) in cortical neurons following 6-h treatment in the indicated conditions. In (c), longer exposure of the membrane was required to visualize the dimeric Complex V. Graphs represent mean and s.e.m of (b)n=5 and (d)n=3 independent experiments. Mon=monomers, Dim=dimers, and CV=Complex V. (e) Representative BN-PAGE of the indicated respiratory complexes using anti-NDUFA9 (Complex-I), anti-ATP5a (Complex-V) and anti-Core2 (Complex-II). Cortical neurons were treated for 6 h in the indicated conditions. SC 1–5=supercomplex assembly. (f) Quantification of relative assembly of supercomplexes visualized using anti-NDUFA9 (Complex-I). Mean and s.e.m ofn=4 independent experiments. (g,h) Representative BN-PAGE of the indicated respiratory complexes using anti-NDUFA9 (Complex-I), anti-UQCRC2 (Complex-III), anti-Complex IV subunit 1 (Complex-IV) and anti-Core2 (Complex-II) following 6 h in the indicated conditions. Graphs in (h) are mean and s.e.m ofn=6 (Complex-I),n=4 (Complex-III) andn=3 (Complex-IV) independent experiments. (i,j)OCR in cortical neurons using a Seahorse XF24 Extracellular Flux Analyzer. Mean and s.d. (n=4 replicates from three independent experiments). *P<0.05; **P<0.01; ***P<0.001 (Student’st-test). Figure 8: Acidosis instigates an adaptive reprogramming of mitochondrial respiratory efficiency. ( a – d ) Representative BN-PAGE of Complex V (ATP synthase) ( a ) monomers (whole cells) and ( c ) dimers (isolated mitochondria) in cortical neurons following 6-h treatment in the indicated conditions. In ( c ), longer exposure of the membrane was required to visualize the dimeric Complex V. Graphs represent mean and s.e.m of ( b ) n =5 and ( d ) n =3 independent experiments. Mo n =monomers, Dim=dimers, and CV=Complex V. ( e ) Representative BN-PAGE of the indicated respiratory complexes using anti-NDUFA9 (Complex-I), anti-ATP5a (Complex-V) and anti-Core2 (Complex-II). Cortical neurons were treated for 6 h in the indicated conditions. SC 1–5=supercomplex assembly. ( f ) Quantification of relative assembly of supercomplexes visualized using anti-NDUFA9 (Complex-I). Mean and s.e.m of n =4 independent experiments. ( g , h ) Representative BN-PAGE of the indicated respiratory complexes using anti-NDUFA9 (Complex-I), anti-UQCRC2 (Complex-III), anti-Complex IV subunit 1 (Complex-IV) and anti-Core2 (Complex-II) following 6 h in the indicated conditions. Graphs in ( h ) are mean and s.e.m of n =6 (Complex-I), n =4 (Complex-III) and n =3 (Complex-IV) independent experiments. ( i , j) OCR in cortical neurons using a Seahorse XF24 Extracellular Flux Analyzer. Mean and s.d. ( n =4 replicates from three independent experiments). * P <0.05; ** P <0.01; *** P <0.001 (Student’s t -test). Full size image The ability of post-mitotic cells to adapt and survive physiological or pathological stress, such as that imposed by oxygen deprivation, has been a long-standing question in biology. Here we report that mild extracellular acidosis, a biological consequence of anaerobic metabolism during hypoxia, restructures the mitochondrial network as an adaptive mechanism to enhance mitochondrial function and promote cellular survival. Mitochondrial remodelling by acidosis, through the activation of a dual programme that modulates mitochondrial dynamics and architecture, represents a novel and physiological pathway that sustains mitochondrial integrity and ATP production despite oxygen limitations. Preventing this reversible and homeostatic process results in mitochondrial dysfunction, fragmentation and cell death. We provide a mechanism underlying the protective nature of mild acidosis, identify a novel physiological regulator of mitochondrial dynamics in post-mitotic cells and propose a role for mitochondrial morphology in the bioenergetic status of cells. Survival of post-mitotic cells is highly dependent on a sufficient supply of energy to uphold the exhaustive demands incurred by complex molecular networks. The switch to anaerobic metabolism, albeit a critical cellular metabolic adaptation of hypoxic cells, cannot compensate for the loss of mitochondrial respiration during prolonged hypoxia [54] , [65] , [66] . As a result, cells faced with prolonged hypoxia will inevitably endure energy failure and cell death if not counteracted with an increase in energy supply. Data presented here demonstrate that post-mitotic cells have evolved a rapid and reversible mechanism to uphold efficient ATP production, via mitochondrial remodelling, that is regulated by acidosis. This is, to our knowledge, the first ascribed function for this metabolic product of anaerobic respiration historically associated with clinical resistance during ischemic insults. We propose a model whereby a threshold accumulation of extracellular protons, acquired through an initial increase in the glycolytic rate during hypoxia, would relay a signal back to mitochondria, potentially via changes in intracellular pH, in order to modulate mitochondrial bioenergetics ( Fig. 9 ). 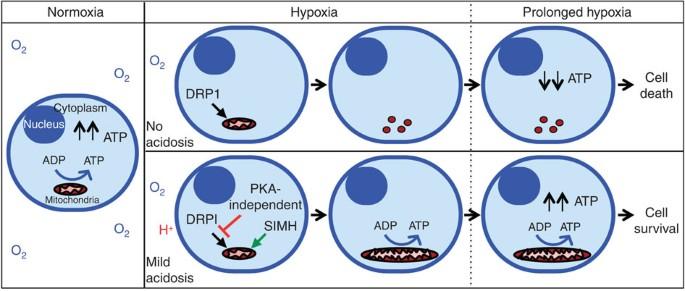Figure 9: Mitochondrial restructuring by mild acidosis determines cellular bioenergetics during hypoxia. The cartoon depicts the cascade of events following a decrease in oxygen levels and the role of mild acidosis in triggering mitochondrial restructuring and reprogramming to determine cellular bioenergetics and cell fate. Upper row: hypoxia causes mitochondrial fragmentation, loss of efficient ATP production and eventual cell death. Lower row: mild acidosis during hypoxia prevents DRP1-mediated fission and promotes mitochondrial elongation (in a SIMH-dependent manner) and cristae remodelling to maintain ATP levels and cell survival. In our model and experiments, ‘no acidosis’ and ‘mild acidosis’ indicate an extracellular pH of 7.2 and 6.5, respectively; ‘hypoxia’ indicates incubation at 1% oxygen for 0–12 h, and ‘prolonged hypoxia’ is considered following 12–21 h of incubation at 1% oxygen. Figure 9: Mitochondrial restructuring by mild acidosis determines cellular bioenergetics during hypoxia. The cartoon depicts the cascade of events following a decrease in oxygen levels and the role of mild acidosis in triggering mitochondrial restructuring and reprogramming to determine cellular bioenergetics and cell fate. Upper row: hypoxia causes mitochondrial fragmentation, loss of efficient ATP production and eventual cell death. Lower row: mild acidosis during hypoxia prevents DRP1-mediated fission and promotes mitochondrial elongation (in a SIMH-dependent manner) and cristae remodelling to maintain ATP levels and cell survival. In our model and experiments, ‘no acidosis’ and ‘mild acidosis’ indicate an extracellular pH of 7.2 and 6.5, respectively; ‘hypoxia’ indicates incubation at 1% oxygen for 0–12 h, and ‘prolonged hypoxia’ is considered following 12–21 h of incubation at 1% oxygen. Full size image In recent years, mitochondrial structure and dynamics have emerged as a fundamental aspect for biological life. Our work further highlights this concept in demonstrating the protective nature of mitochondrial restructuring during stress. In addition, we provide a link between mitochondrial morphology and cristae architecture with the metabolic state of cells. The data presented in this study suggest that mitochondrial remodelling can instigate a systemic reconfiguration of mitochondrial efficiency to extract more ATP per oxygen molecule. In essence, acidosis-mediated reorganization of mitochondrial efficiency can override oxygen limitations and allow for the persistence of mitochondrial respiration in an anaerobic environment. This observation refines the well-established role of oxygen as a limiting factor for oxidative phosphosphorylation and puts forth the idea that mitochondrial reprogramming can dictate the bioenergetics of the cell. In view of these findings, the capability of post-mitotic cells to sense and adapt to anaerobic conditions by inducing anaerobic mitochondrial respiration should emerge as a central research theme in the study of physiological and pathological situations that relates to oxygen and energy homeostasis. Mice, primary neuronal cultures and cell lines To generate dorsal telencephalon-specific MFN1 conditional mutant mice, floxed MFN1 (Jackson Laboratories) and Emx1-cre heterozygous females were bred with floxed MFN1 homozygous and MFN2 heterozygous males. Telencephalon-specific SLP2 conditional mutants were generated by breeding floxed SLP2 homozygous females with Foxg1-cre male mice (provided by Dr Sean Cregan). Cortical neurons were cultured from CD1 wild-type female and male mice (Charles River) and MFN1 or SLP2 conditional knockout mice at embryonic day 14.5 or 15.5 (ref. 67 ). CGNs were cultured from CD1 mice at postnatal day 7 or 8 (ref. 13 ). All experiments were approved by the University of Ottawa’s Animal Care ethics committee adhering to the Guidelines of the Canadian Council on Animal Care. Neurons were maintained in culture for 3–5 days before experimentation. MCF-7 breast carcinoma, A549 lung carcinoma, P19 embryonic teratocarcinoma, Cos7 African green monkey kidney fibroblasts, HeLa and C2C12 myoblasts were obtained from ATCC (Manassas, VA, USA). Primary and transformed MEFs were generated from CD1 mice on embryonic day 13.5. In vitro differentiation of C2C12 myoblasts into multinucleated mytotubes was performed by replacing fetal bovine serum (FBS)-containing DMEM with DMEM containing 2% horse serum when myoblasts were at 80% confluency. Media were changed every second day for about 7 days until multinucleated myotubes were formed. Cell culture The plating density for each cell population was chosen to optimize the rate of physiological extracellular acidification during hypoxic conditions. Cortical neurons and CGNs were seeded on plates (with or without coverslips) coated with 0.01 mg ml −l poly-D-lysine (BD Bioscience) for all experiments. Cortical neurons were plated onto four-well plates, 35- and 60-mm dishes with 4.0 × 10 5 , 3.0 × 10 6 and 9.0 × 10 6 neurons, respectively, and maintained in Neurobasal media (Gibco) that contained 2% B27 (Gibco), 1% N2 (Gibco), 0.6 mM L-glutamine (Gibco) and 1% Pen-Strep (Sigma). CGNs were plated in four- or 12-well plates with 4 × 10 5 and 8 × 10 5 , respectively, and maintained in DMEM (Wisent Inc.) that contained 10% dialysed FBS (Sigma), 25 mM KCl, 2 mM glutamine (Invitrogen), 25 mM glucose and 0.1 mg ml −l gentamycin (Sigma). MCF-7 and MEFs were plated in 35-mm dishes with 7 × 10 5 cells and maintained in DMEM containing 5% FBS and 1% Pen-Strep. All cells were maintained at 37 °C under 5% CO 2 environment until experimentation. Hypoxia was achieved by incubation in a hypoxic chamber at 37 °C under a 1% O 2 , 5% CO 2 and N 2 -balanced atmosphere. Acidosis experiments were conducted as previously described [68] , with modifications. For acidosis experiments mimicking physiological conditions, SD or AP media was utilized. Buffer-free and low glucose (5.5 mM) medium (DMEM; Gibco) was freshly prepared and supplemented with B27 and N2 for post-mitotic neurons or 5% FBS for replicating cells. The level of physiological acidification of the extracellular environment is proportional to the cell density and the buffering capacity of the media. NaHCO 3 was added at 10 mM (post-mitotic cells) or 35 mM (replicating cells) and the pH was adjusted with HCl to 7.2 (SD media) or 6.5 (AP media). Air was bubbled into both media at 22 °C, which stabilizes the pH at 7.2. Culture media were aspirated and cells were washed × 2 in buffer-free low glucose DMEM to remove all traces of highly buffered culture media. Cells were then placed in AP or SD media. AP media slowly reverted to its original set pH under hypoxia, whereas the SD medium remained at pH 7.2. For acute acidosis experiments in hypoxia or normoxia, 30 mM of MES was used as a buffer and the pH was set and stabilized at the required value. Viruses and materials Recombinant adenoviral vectors carrying the DRP1-YFP or GFP expression cassette were prepared using the AdEasy system [12] . Lentivirus vectors carrying photoactivable GFP-ornithine carbamyltransferase (PA-GFP-Oct), Mito-DsRed, shRNA scramble control (shCtr sequence; 5′-CAACAAGATGAAGAGCACCAA-3′), and mouse-specific short-hairpin RNA (shRNA) OPA1 (shOPA1 sequence; 5′-GCCTGACTTTATATGGGAAAT-3′) were prepared using the ViraPower lentiviral expression system (Invitrogen) [13] . For lentiviruses and adenoviruses, neurons were transduced with 2 MOI (multiplicity of infection) or 50–100 MOI, respectively, at time of plating. For all experiments using viruses, neurons were infected with adenovirus or lentivirus for 72 h before experimentation. Oligomycin (10 μM), 6-deoxyglucose (6-DOG, 6 mM), cycloheximide (100 μg ml −l ), CPT (20 μM), mdivi-1 (50 μM), H89 (20 μM), forskolin (25 μM) and Monensin (1 μM) were used where indicated. Immunofluorescence Cells seeded on coverslips were fixed with 4% paraformaldehyde in PBS for 20 min at room temperature. Primary antibodies used were Tom20 (Santa Cruz; 1:100), Tuj1 (Covance; 1:10,000), MAP2 (Novus Biologicals; 1:200), NeuN ( Millipore; 1:1,000), DLP1 (BD Biosciences; 1:100), Cytochrome c (BD Biosciences; 1:100) and Bax (Santa Cruz, 1:100). Cells were incubated for 1 h with a primary antibody solution containing 1% bovine serum albumin (BSA), 0.1% Triton-X-100 in PBS. Cells were washed several times in PBS before 1-h incubation with a secondary 594 or 488 Alexa (Invitrogen; 1:400). Hoechst stain 33342 (Sigma) or 4',6-diamidino-2-phenylindole (DAPI) was added to visualize nuclei and coverslips were mounted using Immunomount (Thermo Scientific). Immunohistochemistry Coronal hippocampal slice preparations (200 μm) were incubated in oxygenated artificial cerebrospinal fluid (ACSF) buffered with PIPES to pH 7.2 or 6.5 for 4 h. Hippocampal slices were fixed for 20 min with ice-cold 4% paraformaldehyde in 1 × PBS and then rinsed twice with 1 × PBS. Slices were incubated in 10% sucrose and embedded in OCT and then sectioned using a microtome to 15-μm sections. Sections were stained with primary antibodies specific to Tom20 and NeuN in 10% normal goat serum-0.1% TritonX/0.1% Tween-20 in PBS overnight at 4 °C followed by 3 × 5 min washes with 1 × PBS. Sections were incubated with secondary antibodies in PBS for 1 h, washed for 5 min, stained with DAPI for 5 min, and then washed with 1 × PBS for 3 × 5 min. Slides were mounted using Immunomount (Thermo Scientific). Representative samples were imaged using a Zeiss Axiovert 100 (Oberkochen, Germany) confocal microscope equipped with a QiCam Digital camera (QImaging Corporation) and Zen software. Mitochondrial length Mitochondrial length was assessed by staining with Tom20 (translocase of outer mitochondria). Mitochondrial length was measured by tracing the mitochondria using the ImageJ software. Mitochondrial length was either binned into different categories (<0.5 μm, 0.5–1 μm, 1–2 μm, >2 μm) or taken as an average. Intracellular pH measurements Changes in intracellular pH was determined utilizing the ratiometric fluorescent intracellular pH indicator BCECF-AM (Invitrogen). Intracellular pH measurements were performed on cultured cortical neurons plated in 96-well black microplates that were treated for 6 h in the appropriate experimental media and subsequently loaded with BCECF-AM (1 μM) for 30–45 min at 37 °C. A dual-excitation ratio of 480 and 440 nm and fixed emission at 535 nm was used to measure changes in BCECF-AM fluorescence. Since these experiments were designed to determine the effect of extracellular acidosis on intracellular pH, the measurements had to be performed while the cells were maintained in the respective experimental media (that is, media at pH 7.2 or pH 6.5). For this reason, the use of BCECF-AM was first validated by performing a calibration curve, using the high K+ Nigericin technique, to ensure that intracellular changes in pH can be detected in the experimental media. MES-buffered DMEM media was supplemented with 130 mM KCl and the pH was set to 6.0, 6.5, 7.0, 7.5 and 8.0 using KOH. The media of cells previously loaded with BCECF-AM (for 30–45 min) was replaced with the high K+ MES-buffered media supplemented with the ionophore Nigericin (Molecular Probes, 10 μM) and incubated for 10 min to allow for equilibration of the intracellular pH with the controlled extracellular medium. BCECF-AM fluorescence was measured as described above. Immunoblot For total cell lysates, cells were washed with PBS, lysed with 4% SDS in PBS, boiled for 5 min and the DNA was sheared by passage through a 26-gauge needle. Primary antibodies recognizing Complex I subunit NDUFA9 (Invitrogen; 1:1,000), Complex II 70-KDa Fp subunit (Invitrogen; 1: 10,000), ATP5a (Abcam; 1:1,000), Complex IV subunit 1 (Invitrogen; 1:1,000), Complex III core protein 2 (UQCRC2, Abcam; 1:1,000), DLP1 (DRP1, BD Transduction Laboratories; 1:1,000), Phoso-DRP1 S637 and S616 (Cell Signaling; 1:1,000), Fis1 (Biovision; 1:500), OPA1 (Abcam; 1:1,000), MFN1 and 2 (Abcam; 1:1,000), VDAC (Abcam; 1:1,000), mitochondrial heat-shock protein 70 (mtHSP70, Thermo Scientific; 1:5,000) and Actin (Santa Cruz; 1:1,000) were used. A secondary antibody conjugated to horseradish peroxidase (Jackson ImmunoResearch) was used and detected using Western Lightning Chemiluminescence Reagent Plus (Perkin Elmer). Representative full-gel bots are shown in Supplementary Fig. 17 . Immunoprecipitation Cells were lysed in RIPA buffer (50 mM Tris (pH 7.2), 150 mM NaCl, 10% NP40 and 1 mM sodium orthovanadate with a protease inhibitor cocktail (PIC)). Cell lysates were incubated with anti-DRP1 antibody (BD Transduction Laboratories) for 1 h while tumbling at 4 °C, followed by overnight incubation with Sepharose A/G beads blocked in 2% BSA. Beads were washed 4 × in 1 × Tris-buffered saline and eluted by boiling at 95 °C for 4 min. Time-lapse imaging and mitochondrial fusion assay Cortical neurons were seeded on 35-mm dishes with coverslip bottoms (MatTek) coated with poly-D-lysine (VWR International) and infected with 2 MOI of the photoactivable GFP tagged to ornithine carbamyltransferase (PA-GFP-Oct) and Mito-DsRed. Following 2-h incubation in MES-buffered media at pH 7.2 or 6.5, plates were mounted in a temperature-controlled chamber (37 °C) and visualized with an LSM-510 confocal laser-scanning microscope (Axiovert 200), with a × 63 oil immersion objective. Mitochondrial fusion assays were performed as described previously with modifications [13] . Briefly, PA-GFP-Oct was first pre-imaged and scanned to ensure that there is no spontaneous activation. PA-GFP-Oct was then photoactivated with a 405-nm laser and the spreading of the signal was imaged every 2 min using a 488-nm line for a total of 22 min. Mito-DsRed was excited at 543 nm and was used a guide to ensure that the ROI for PA-GFP-Oct activation was within the mitochondria. The fusion rate was expressed as a relative measure of pixel intensity at the indicated time over that at t =0 min (where 0 min represents the signal detected after 2 min of photoactivation and equilibration of GFP signal). OPA1 crosslinking In vivo crosslinking reactions were performed at 37 °C with 10 mM BMH crosslinker (Fisher Scientific) for 20 min. Reactions were terminated by adding 0.001% β-mercaptoethanol. Cells were lysed following crosslinking, and analysed by gradient gel electrophoresis using NuPAGE Novex 3–8% Tris-acetate gradient gels (Life Technologies), followed by western blotting against OPA1. (TEM) and cristae analyses Mitochondrial ultrastructure was analysed from whole cells of cultured cortical neurons following 6-h treatment in the appropriate conditions. Briefly, plated neurons were rapidly washed in PBS and harvested by scraping very lightly. Neurons were fixed in 2% gluteraldehyde for 20 min at room temperature and stored immediately at 4 °C for processing as previously described [69] . Cristae analysis was performed using ImageJ and a minimum of 100 mitochondria were analysed. For each individual cristae, the average diameter was measured from three representative regions. Cytochrome c release Neurons were treated with 20 μM CPT for the indicated times, fixed and stained with cytochrome c and Tom20-specific antibodies. For each replicate, a total of 100 neurons were counted from three to five different fields using a Zeiss 510 meta confocal microscope. A diffused cytochrome c staining or complete lack of staining was identified as release. Cell viability assay Following 30 h of incubation under the indicated conditions, cells were subjected to a live–dead assay (Invitrogen) by staining with calcein (live cells) and ethidium homodimer-1 (dead cells) for 10–15 min at 37 °C. In each replicate, three to five different fields were randomly chosen and imaged per treatment group. Cell death was expressed as a percentage of total cells. Calcein and ethidium homodimer-1 dyes are unaffected by pH as neutralization of an acidic set or acidification of a neutral set immediately before addition of the dyes yielded the same results. Mitochondrial membrane potential Neurons were seeded in 96-well black microplates. Following the appropriate treatment, 50 nM TMRE was added and cells were incubated for 30 min at 37 °C under normoxia (control) or hypoxia. FCCP (1 μM) was added to the appropriate wells 10 min before addition of TMRE. Neurons were washed in PBS and TMRE fluoresence was measured in a plate reader at Ex 510 nM an Em 590 nM. ATP assay ATP concentrations were measured with the CellTiter-Glo Luminescent Assay (Promega) using a LUMIstar Galaxy luminometer (BMG Labtechnologies) according to the manufacturer’s protocol. Data were collected from multiple replicate wells for each experiment. Viability of cells under all conditions was ensured by PI staining. Blue-native PAGE ETC supercomplexes and ATP synthase assembly were analysed from whole cells or isolated mitochondria [70] . For whole cells, following the indicated treatments, cells were harvested in PBS on ice, pelleted at 960 g for 5 min at 4 °C. For isolated mitochondria, cells were washed with PBS and lysed in mitochondrial isolation buffer (200 mM mannitol, 70 mM sucrose, 10 mM HEPES, pH 7.4, 1 mM EGTA, PIC 1:1,000) on ice using a 25-G needle. Following centrifugation at 110 g for 9 min to remove nuclei and cellular debris, the supernatant was centrifuged at 8,600 g for 9 min to pellet mitochondria. This differential centrifugation step was repeated to further purify the mitochondrial fraction. For BN-PAGE analysis, pellets of whole cells or isolated mitochondria were resuspended in digitonin extraction buffer (50 mM imidazole/HCl pH 7.0, 50 mM NaCl, 5 mM 6-aminohexanoic acid, 1 mM EDTA and the appropriate ratio of digitonin). A 1% digitonin ratio was used for Complex-1 and supercomplexes, and 2% was used for ATP synthase assembly. One hundred fifty micrograms were loaded with 5% glycerol and 1:10 dye:digitonin ratio of coomassie dye in 500 mM 6-aminohexanoic acid on 3–13% large acrylamide gradient gels. Gels were transferred to nitrocellulose membranes and the resulting membranes were subjected to immunoblotting. Oxygen consumption The Seahorse XF24 Extracellular Flux Analyzer (Seahorse Biosciences; North Billerica, MA, USA) was used to measure oxygen consumption in cells. Cortical neurons were seeded onto 24-well Seahorse plates at a density of 1.5 × 10 5 cells per well. Following treatment, cells were washed with modified Kreb’s Ringer Buffer (128 mM NaCl, 4.8 mM KCl, 1.2 mM KH 2 PO 4 , 1.2 MgSO 4 , 25 mM CaCl 2 , 0.1% BSA (fatty acid-free), 10 mM glucose and 1 mM sodium pyruvate, pH 7.4) and placed in Kreb’s Ringer Buffer for 15 min at 37 °C before loading into the XF Analyser. Following mesurements of resting respiration, cells were treated sequentially with the following: oligomycin (0.2 μg μl −l ), to measure the nonphosphorylating OCR; FCCP (1 μM), to get the maximal OCR; and antimycin A (2.5 μM) and rotenone (1 μM), to measure the extramitochondrial OCR. Each measurement was taken over a 2-min interval followed by 2 min mixing and 2 min incubation. Three measurements were taken for the resting OCR, three after oligomycin treatment, two after FCCP and two after antimycin A and rotenone. Quantification and statistical analysis For mitochondrial length measurements, all mitochondria in a field were measured as per condition and a minimum of 1,000 mitochondria were measured for each treatment. For cell death studies, a minimum of 300 cells per field (minimum five fields) were scored for each treatment at the indicated time points. The data represent mean values±s.d. from three independent experiments ( n =3) unless otherwise noted. P -values were obtained using a two-tailed Student’s t- test. How to cite this article: Khacho, M. et al. Acidosis overrides oxygen deprivation to maintain mitochondrial function and cell survival. Nat. Commun. 5:3550 doi: 10.1038/ncomms4550 (2014).